Relative motions between left flipper and dorsal fin domains favour P2X4 receptor activation Channel gating in response to extracellular ATP is a fundamental process for the physiological functions of P2X receptors. Here we identify coordinated allosteric changes in the left flipper (LF) and dorsal fin (DF) domains that couple ATP-binding to channel gating. Engineered disulphide crosslinking or zinc bridges between the LF and DF domains that constrain their relative motions significantly influence channel gating of P2X4 receptors, confirming the essential role of these allosteric changes. ATP-binding-induced alterations in interdomain hydrophobic interactions among I208, L217, V291 and the aliphatic chain of K193 correlate well with these coordinated relative movements. Mutations on those four residues lead to impaired or fully abolished channel activations of P2X4 receptors. Our data reveal that ATP-binding-induced altered interdomain hydrophobic interactions and the concomitant coordinated motions of LF and DF domains are allosteric events essential for the channel gating of P2X4 receptors. P2X receptors are ATP-gated ion channels, and the opening of P2X receptors in response to extracellular (EC) ATP is a fundamental process in signal transduction in both excited and non-excited cells [1] . The delineation of ATP-binding, allosteric conformational changes in EC domains, together with pore dynamics correlated to channel gating, will promote the development of new pharmacological agents for P2X receptors [2] , [3] . Recently, the solution of crystal structures of the zebra fish P2X4 (zfP2X4, PDB entry codes: 3H9V and 4DW1) receptor in the presence and absence of ATP provided an insight into the architecture of the ATP-binding site and the ion channel pore, together with the conformational changes associated with channel gating [4] , [5] . Those structures confirm the predicted topology of P2X receptors that contains a large, glycosylated and disulphide-rich EC domain, two transmembrane (TM) domains and N- and C-intracellular termini [3] , [4] , [5] . The architecture of P2X receptors resembles the shape of a dolphin [4] , [5] , containing a rigid central EC body domain, which is attached by the structurally different head, left flipper (LF), right flipper (RF) and dorsal fin (DF) domains. Numerous studies have demonstrated that a downward motion of the cysteine-rich head domain, tightening of the ATP-binding site jaw and upper vestibule expansion are essential for activation, desensitization and sustained activation of P2X receptors [5] , [6] , [7] , [8] , [9] , [10] , with data obtained from the application of multiple approaches, including electron microscopy [10] , voltage-clamp fluorometry [9] , engineering EC metal bridges [8] , [11] , normal mode analysis (NMA) [7] , molecular dynamics (MD) simulations [7] and fast-scanning atomic force microscopy [6] . Those studies provide new insights into the dynamics of EC domain as well as the movements of the whole receptor during channel gating. Notably, a more pronounced deformation of the EC domain was observed in biophysical, biochemical and computational analysis of the P2X receptor than that observed in ATP-bound open structure, especially for the head domain and the upper vestibule [6] , [10] . These apparently less pronounced allosteric conformational changes may be attributable to different data from distinct subunits of P2X receptors. In addition, the possibility that the crystallization conditions have an effect [12] on the native conformation of zfP2X4 cannot be completely excluded. Making further explorations on the allosteric changes of EC domain will contribute to our understanding of the nature and extent of ATP-binding-induced conformational changes on channel activation of this distinct family of trimeric ligand-gated ion channels. Besides the head domain, the open structure of zfP2X4 also suggests that LF and DF domains undergo conformational changes during channel activation [5] . However, whether those allosteric changes are essential for channel activation or not and how ATP-binding contributes to allosteric changes of those two domains remain unclear. Taking advantage of the known crystal structures of closed and open states, and with the use of a multidisciplinary approaches including molecular modelling, site-directed mutagenesis, electrophysiology, protein expression analysis, engineered disulphide crosslinking and engineered zinc bridge, here we uncover key residues involved in ATP-binding-induced coordinated movements of LF and DF domains, and demonstrate the essential role of those relative motions in channel gating of P2X4 receptors. Structural dynamics of LF and DF domains during simulations The closed structure [4] of zfP2X4 outlined the static architecture of this ion channel ( Supplementary Fig. 1a ). To further illustrate the inherent structural dynamics at the atomic level as well as the correlation between the dynamics and channel activation, a 300-ns MD simulation was carried out under conditions in which the effects of temperature (300 K), water and membrane on channel dynamics were adequately considered. Root mean square deviation calculations indicated that it took ~40–50 ns for this structure to attain the equilibrium state ( Supplementary Fig. 1b ), a period that is significantly longer than that of one of structurally similar trimeric channels [13] , that is, the ASIC3 channel [14] . This implied that the zfP2X4 receptor underwent significant structural rearrangements under normal temperature and pH conditions during the timescale of the MD simulations ( Supplementary Movie 1 ). A superposition and comparison of the initial and the equilibrated representative conformation after MD simulations confirmed the structural dynamics of zfP2X4 at the room temperature in the absence of ATP, especially for β 12-13 , head, LF and DF domains ( Fig. 1a and Supplementary Movie 1 ). Surprisingly, the integrated structural rearrangements of these domains resulted in a spontaneous closure of the ATP-binding site jaw ( Fig. 1b and Supplementary Movie 1 ), and an expansion of the upper vestibule ( Fig. 1c , Supplementary Fig. 1c and Supplementary Movie 1 ). Those structural changes are widely accepted to associate with channel opening [6] , [7] , [8] , [10] . Nevertheless, a comparison of pore size of the initial and representative conformation after MD simulations ( Fig. 1c ), and continuous pore-size measurements ( Supplementary Fig. 1d ) revealed that there was no obvious dilation of the TM pore observed even though these open-related structural events had taken place. These observations confirmed the essential role of inherent dynamics in favouring the tightening of ATP-binding site jaw as well as the expansion of the upper vestibule. Meanwhile, these results also implied that other open-related allosteric changes may be curbed because of the absence of ATP during MD simulations. 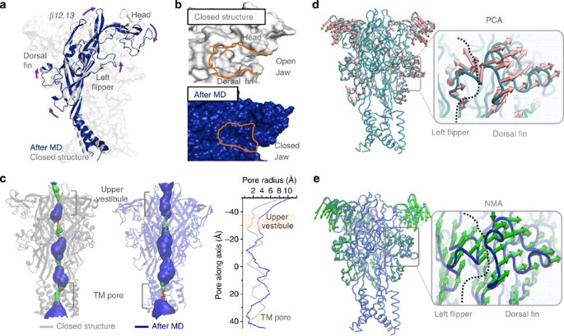Figure 1: Inherent dynamics of zfP2X4 in the absence of ATP. (a–c) Superposition of the initial (grey, PDB ID code 3H9V) and representative equilibrated structure (blue) after 300-ns MD simulations on closed zfP2X4 structure. Significant structural alterations in β12-13, head, LF and DF domains (a), the spontaneous closure of the ATP-binding jaw (b), and the expansion of upper vestibule (c) occurred during 300-ns MD simulations. (d,e) Vector representation of the motions of LF and DF domains in principal component analysis (PCA) (d) and intrinsic dynamics of NMA mode (e) of zfP2X4. The movements of LF and DF domains were highlighted within enlarged rectangular box. The vector arrows represent both the amplitudes and directions of the displacements experienced by residues during conformational changes. Dotted lines denote the interface of LF and DF domains. Figure 1: Inherent dynamics of zfP2X4 in the absence of ATP. ( a – c ) Superposition of the initial (grey, PDB ID code 3H9V) and representative equilibrated structure (blue) after 300-ns MD simulations on closed zfP2X4 structure. Significant structural alterations in β 12 - 13 , head, LF and DF domains ( a ), the spontaneous closure of the ATP-binding jaw ( b ), and the expansion of upper vestibule ( c ) occurred during 300-ns MD simulations. ( d , e ) Vector representation of the motions of LF and DF domains in principal component analysis (PCA) ( d ) and intrinsic dynamics of NMA mode ( e ) of zfP2X4. The movements of LF and DF domains were highlighted within enlarged rectangular box. The vector arrows represent both the amplitudes and directions of the displacements experienced by residues during conformational changes. Dotted lines denote the interface of LF and DF domains. Full size image As revealed by a superposition of the initial and the equilibrated representative conformations ( Fig. 1a ) as well as a continuous measurement of C α –C α distances between zf P125 (head; the superscript ‘zf’ denotes zfP2X4 numbering, similarly hereinafter), zf V291 (LF) and zf H219 (DF) in MD simulations ( Supplementary Fig. 2a,b,e,f ), both the LF and DF domains underwent upward movements and came closer to the head domain when bound ATP is absent in MD simulations. Principal component analysis (PCA) of snapshots from MD simulations ( Fig. 1d ) or a low-frequency dynamics mode derived from NMA of the closed structure ( Fig. 1e and Supplementary Movie 2 ) confirmed the tendency of upward motions of both the LF and DF domains in the absence of ATP. Interestingly, those movements are distinct from an upward motion of the DF domain and a downward motion of the LF domain observed in the ATP-bound open crystal structure of zfP2X4 ( Fig. 2a ). In addition, the relative motions with a downward motion of the LF domain and an upward motion of the DF domain were also observed in another set of MD simulation on the closed zfP2X4 structure complexes with pre-docked ATP (see below). These data indicated that the bound ATP might break the inherent dynamics of LF and DF domains, which has an essential role in channel gating of P2X4 receptors. 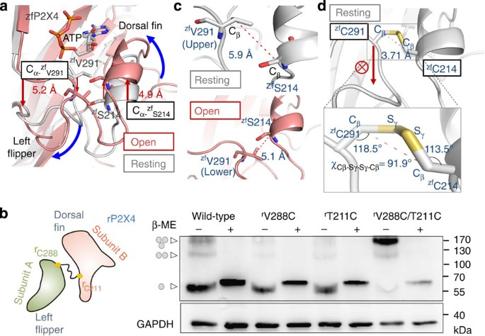Figure 2: Disulphide crosslinking between LF and DF constrains the relative motion of LF and DF domains. (a) A superposition of the closed (grey, PDB ID code 3H9V) and open (pink, PDB ID code 4DW1) structures of zfP2X4. Blue arrows denote movements of LF and DF domains from the closed state to the ATP-bound open state. Red arrows indicate the relative movements of Cαatoms ofzfV291 andzfS214 from the closed state to the open state. (b) Interdomain/intersbunit disulphide bond betweenrV288C andrT211C in the homooligomeric rat P2X4 (rP2X4) receptor. Wild-type rP2X4,rV288C,rT211C andrV288C/T211C subunits (each carrying a C-terminal EE epitope) were transiently expressed in HEK-293 cells. Cells were lysed in buffers with or without β-ME (1%, 10 mM) as indicated. Protein samples were separated on SDS-PAGE gels and detected by western blotting via an anti-EE antibody. The band indicated by arrowheads corresponds to the expected size of the monomeric, dimer and trimetric rP2X4 subunits, respectively; protein molecular weight markers are indicated on right. These results were observed in at least three independent experiments for each receptor. (c) The locations ofzfV291 andzfS214 in the resting (upper) and open (down) structures of zfP2X4. Red dashed line indicates the measured Cβ–Cβdistance betweenzfV291 andzfS214. (d) Zoom-in view of constructed disulfide-bridge model of zfP2X4V291C/S214Cbased on the closed structure showing details of Cβ–Cβdistance (red dashed line) and the dihedral angle measured between Cβ–Sγ–Sγ–Cβatoms from thezfC291 andzfC214. Figure 2: Disulphide crosslinking between LF and DF constrains the relative motion of LF and DF domains. ( a ) A superposition of the closed (grey, PDB ID code 3H9V) and open (pink, PDB ID code 4DW1) structures of zfP2X4. Blue arrows denote movements of LF and DF domains from the closed state to the ATP-bound open state. Red arrows indicate the relative movements of C α atoms of zf V291 and zf S214 from the closed state to the open state. ( b ) Interdomain/intersbunit disulphide bond between r V288C and r T211C in the homooligomeric rat P2X4 (rP2X4) receptor. Wild-type rP2X4, r V288C, r T211C and r V288C/T211C subunits (each carrying a C-terminal EE epitope) were transiently expressed in HEK-293 cells. Cells were lysed in buffers with or without β-ME (1%, 10 mM) as indicated. Protein samples were separated on SDS-PAGE gels and detected by western blotting via an anti-EE antibody. The band indicated by arrowheads corresponds to the expected size of the monomeric, dimer and trimetric rP2X4 subunits, respectively; protein molecular weight markers are indicated on right. These results were observed in at least three independent experiments for each receptor. ( c ) The locations of zf V291 and zf S214 in the resting (upper) and open (down) structures of zfP2X4. Red dashed line indicates the measured C β –C β distance between zf V291 and zf S214. ( d ) Zoom-in view of constructed disulfide-bridge model of zfP2X4 V291C/S214C based on the closed structure showing details of C β –C β distance (red dashed line) and the dihedral angle measured between C β –S γ –S γ –C β atoms from the zf C291 and zf C214. Full size image Disulphide crosslinking between LF and DF domains To test this idea, we constrained the relative motions between LF and DF domains by introducing cysteine residues [15] that can form interdomain disulphide bridge ( Fig. 2b ). Owing to the low potency of ATP on the zfP2X4 receptor expressed in mammalian HEK-293 cells [5] , all mutagenesis, electrophysiological recording and protein expressions measurements were carried out on identical residues of rat P2X4 (rP2X4), although the molecular modelling was based on the crystal structures of zfP2X4. Cysteine-scanning mutagenesis in the LF and DF domains of the rP2X4 receptor has identified two positions, r V288 and r T211 (corresponding to zf V291 and zf S214 in zfP2X4, respectively; the superscript ‘r’ denotes rP2X4 numbering, similarly hereinafter; Fig. 2a ), and when both are substituted by cysteine could form an interdomain/intersubunit disulphide bond ( Fig. 2b ). The wild-type rP2X4, and single mutants r V288C and r T211C, migrated on SDS-PAGE gels predominantly at position expected for the monomer subunit (~57 kDa; Fig. 2b ). In contrast, no obvious monomeric form was observed for the subunit containing cysteine at both positions ( r V288C/T211C; Fig. 2b ). The observed higher molecular mass protein presumably represents a disulphide bond trimer, because β-mercaptoethanol (β-ME, 1%) reduced it to a monomeric size. β-ME also caused a modest shift of wild-type subunit or subunits with single cysteine substitution ( Fig. 2b )owing to its effect on the large number of native cysteine residues within EC domain, which is also observed in another subtype of P2X receptors [16] . Nevertheless, it can be reasonably inferred that an intersubunit/interdomain disulphide is formed between the LF and DF domains in the double cysteine mutant r V288C/T211C. The C β –C β distance between identical residues of zfP2X4, zf V291 and zf S214, was slightly reduced in open state (5.1 Å) compared with that of resting state (5.9 Å) ( Fig. 2c ). The C α atom of zf V291 moved downwards ~5.2 Å and the C α atom of zf S214 moved upwards ~4.9 Å along with relative motions between LF and DF domains ( Fig. 2a ; red arrows). Those relative movements led to a final ‘translocation’ between zf V291 and zf S214 ( Fig. 2a,c ). Based on closed crystal structure of zfP2X4, the predicted C β –C β distance of two cysteine residues of zfP2X4 C291/C214 was reduced to ~3.71 Å ( Fig. 2d ). The predicted dihedral angle χ between the C β –S γ –S γ –C β atoms of zf C291 and zf C214 based on the closed crystal structure of zfP2X4) is 91.9° ( Fig. 2d ), a value very close to that of crystal structures ( χ Cβ-Sγ-Sγ-Cβ =±90 o ) [17] . During MD simulations, the predicted dihedral angle χ and C β –C β distance based on the closed structure were stabilized at ~90° and ~3.8 Å ( Supplementary Fig. 3b ). In contrast, the predicted dihedral angle χ and C β –C β distance of zf V291C/S214C based on the open crystal structure of zfP2X4 markedly drifted from the original values during MD simulations (83.5° and 4.09 Å, Supplementary Fig. 3a ), resulting in more obvious spontaneous structural rearrangements in the LF and DF domains ( Supplementary Fig. 3f ) than wild type ( Supplementary Fig. 3e ). Thus, the disulphide bridge between the LF and DF domains would be more compatible with the closed state rather than the open state, and will stabilize the conformation of those two domains in the closed sate. This means that the dihedral angle χ between C β –S γ –S γ –C β atoms of zfC291 and zfC214 would help to block the ‘translocation’ of zfC291 and zfC214, as well as relative motions between LF and DF domains during channel gating. As a result, after expression in HEK-293 cells, the mutated channel of containing cysteine at both positions ( r V288C/T211C) produced a smaller response to ATP (147±47 pA, n =11), when compared with channel carrying single substitutions r T211C (3833±731 pA, n =4) or r V288C (427±73 pA, n =8). The current of r V288C/T211C increased ~2–5 folds after dithiothreitol (DTT) application ( Fig. 3a,c ; n =9); the current declined again after treatment with H 2 O 2 ; the second application of DTT could increase the current of r V288C/T211C again, suggesting that an interdomain disulphide formation between r V288C and r T211C impaired channel gating of rP2X4. Since DTT slightly decreased rather than increased ATP currents in HEK-293 cells expressing wild-type rP2X4 receptor ( Fig. 3b,c ; n =12), the breaking of disulphide bond between r V288C and r T211C may be responsible for the DTT-application-evoked increases in current amplitude of r V288C/T211C. The disulphide crosslinking between C288 and C211 decreased the apparent ATP affinity of r V288C/T211C (EC 50 , the concentration of ATP yielding a current that is half of the maximum, 31.4±13.7 μM, n H=1.74±0.3, and 6.44±2.5 μM, n H=1.78±0.16, for before and after DTT applications, respectively; mean±s.e.m. of EC 50 values derived from 4–6 independent measurements; Fig. 3d,e ), indicating that the relative motions between LF and DF domains were correlated with ATP-sensing of P2X4 receptors. However, the DTT application is also capable of potentiating the saturated ATP (0.3–1 mM)-induced current of rP2X4 receptors ( Fig. 3d,e ), suggesting that the relative motions between LF and DF domains are also essential allosteric changes that couple ATP-binding to channel activation. Those data suggested that the free relative motions between the LF and DF domains are pivotal for ATP-evoked activation of P2X4 receptors. 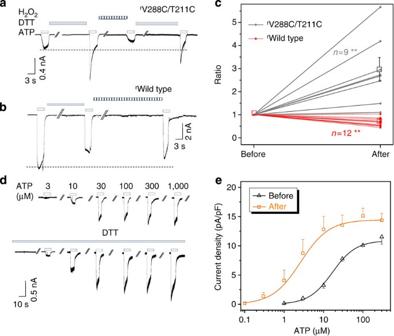Figure 3: Disulphide crosslinking between LF and DF impairs the activation of P2X4 receptors. (a,b) Representative current recordings from cells expressingrV288C/T211C (a), and wild-type rP2X4 (b). Cells were voltage clamped at −60 mV, and currents were evoked by ATP (10 μM, 3 s) at 2 min intervals. Cells were perfused with dithiothreitol (DTT; 10 mM) and H2O2(0.3%) at the times indicated. (c) Pooled data from the combination of experiments ina,b.yaxis stands for the ratio of ATP-evoked currents after DTT treatments normalized by the currents before DTT treatment. Each line represents one paired measurements of an individual cell. Open boxes indicates mean±s.e.m.,n=9–12; **P<0.01 after versus before DTT treatment, pairt-test. (d,e) Effects of disulphide crosslinking on the ATP-sensitivity of rP2X4V288C/T211C. Representative current recordings (d) and pooled data (e) from cells expressing rP2X4V288C/T211Cshow ATP-sensitivity of this double mutant before and after DTT treatments. Concentration–response relationship for ATP activation of rP2X4V288C/T211Cwas obtained by measuring currents in response to different concentrations of ATP and all of the results used to generate a concentration–response relationship before and after DTT treatments were from the same group/cell by using amphotericin-perforated patch clamp. Data points are presented as mean±s.e.m. of 5–8 measurements, and the solid line are fit to Hill equation. The EC50andnH values of ATP for rP2X4V288C/T211Cin the absence and presence of DTT are 31.4±13.7 μM,nH=1.74±0.3, and 6.44±2.5 μM,nH=1.78±0.16, respectively. Figure 3: Disulphide crosslinking between LF and DF impairs the activation of P2X4 receptors. ( a , b ) Representative current recordings from cells expressing r V288C/T211C ( a ), and wild-type rP2X4 ( b ). Cells were voltage clamped at −60 mV, and currents were evoked by ATP (10 μM, 3 s) at 2 min intervals. Cells were perfused with dithiothreitol (DTT; 10 mM) and H 2 O 2 (0.3%) at the times indicated. ( c ) Pooled data from the combination of experiments in a , b . y axis stands for the ratio of ATP-evoked currents after DTT treatments normalized by the currents before DTT treatment. Each line represents one paired measurements of an individual cell. Open boxes indicates mean±s.e.m., n =9–12; ** P <0.01 after versus before DTT treatment, pair t -test. ( d , e ) Effects of disulphide crosslinking on the ATP-sensitivity of rP2X4 V288C/T211C . Representative current recordings ( d ) and pooled data ( e ) from cells expressing rP2X4 V288C/T211C show ATP-sensitivity of this double mutant before and after DTT treatments. Concentration–response relationship for ATP activation of rP2X4 V288C/T211C was obtained by measuring currents in response to different concentrations of ATP and all of the results used to generate a concentration–response relationship before and after DTT treatments were from the same group/cell by using amphotericin-perforated patch clamp. Data points are presented as mean±s.e.m. of 5–8 measurements, and the solid line are fit to Hill equation. The EC 50 and n H values of ATP for rP2X4 V288C/T211C in the absence and presence of DTT are 31.4±13.7 μM, n H=1.74±0.3, and 6.44±2.5 μM, n H=1.78±0.16, respectively. Full size image Engineered zinc bridge between LF and DF domains To further confirm the crucial role of the relative motion of the LF and DF domains in channel activations, we introduced an engineered zinc bridge into the mutated P2X4 receptor containing histidine residues at those two positions. The zinc-bridge model of zfP2X4 V291H/T214H based on the closed crystal structure of zfP2X4 was constructed as previously described [8] (see Methods section). The distance (2.17 Å) and angle (107.7°) between the Zn 2+ and coordinating atom NE2 of histidine residues ( Fig. 4a ) were very close to those obtained from the analysis of 111 crystal structures [18] . The zinc-bridge model of zfP2X4 V291H/T214H based on the open crystal structure also produced reasonable values for the bond angle (110.2°) and bond lengths (2.14 Å; Supplementary Fig. 3c ). However, the predicted model of the metal bridge between the LF and DF domains based on the open crystal structure was less stable during MD simulations when compared with the model based on the closed crystal structure ( Supplementary Fig. 3d ). During 50-ns MD simulations, the C β –C β distance and dihedral angles χ 1 (along C α –C β ) of zf V291H and zf S214H were significantly altered, indicating that the zinc bridge may be not compatible with the open structure of zfP2X4. Similarly, the marked spontaneous structural rearrangements of LF and DF domains after such timescale of MD simulations were observed in zf V291H/S214H ( Supplementary Fig. 3f ) but not in the open structure of wild-type zfP2X4 ( Supplementary Fig. 3e ). Therefore, the zinc bridge between zf H291 and zf H214 would mimic the role of the disulphide crosslinking by constraining the relative motions between LF and DF domains through coordination bonds NE2–Zn–NE2 and the increased C β –C β distance (7.28 Å) between zf H291 and zf H214 ( Fig. 4a ). 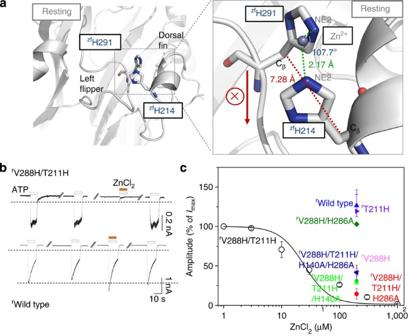Figure 4: Zinc bridge between LF and DF domains blocks channel activation of P2X4 receptors. (a) Zoom-in view of constructed zinc-bridge model of zfP2X4V291H/S214Hbased on the closed structure showing the details of the Cβ–Cβdistance between two histidines (red dotted line), and the distance (green dotted line) and angle measured between Zn2+and coordinating NE2 atoms fromzfH291 andzfH214. (b,c) Examples (b) and summary (c) effects of EC Zn2+on ATP (100 μM, saturating)-evoked current of wild-type and mutated rP2X4 receptors. EC Zn2+(200 μM, saturating) inhibited ATP-evoked currents of mutantsrV288H/T211H,rV288H/T211H/H40A, V288H/T211H/H40A/H286A, V288H/T211H/H286A andrV288H, but slightly potentiated ATP-evoked currents ofrT211H,rV288H/H286A and wild-type rP2X4 receptors. The dose–response curve of Zn2+inrV288H V288H/T211H is fit to Hill1 equation (solid line, IC50=25.6±5.7 μM,nH=−0.97±0.1). Data points are mean±s.e.m. of 3–6 measurements. Figure 4: Zinc bridge between LF and DF domains blocks channel activation of P2X4 receptors. ( a ) Zoom-in view of constructed zinc-bridge model of zfP2X4 V291H/S214H based on the closed structure showing the details of the C β –C β distance between two histidines (red dotted line), and the distance (green dotted line) and angle measured between Zn 2+ and coordinating NE2 atoms from zf H291 and zf H214. ( b , c ) Examples ( b ) and summary ( c ) effects of EC Zn 2+ on ATP (100 μM, saturating)-evoked current of wild-type and mutated rP2X4 receptors. EC Zn 2+ (200 μM, saturating) inhibited ATP-evoked currents of mutants r V288H/T211H, r V288H/T211H/H40A, V288H/T211H/H40A/H286A, V288H/T211H/H286A and r V288H, but slightly potentiated ATP-evoked currents of r T211H, r V288H/H286A and wild-type rP2X4 receptors. The dose–response curve of Zn 2+ in r V288H V288H/T211H is fit to Hill1 equation (solid line, IC 50 =25.6±5.7 μM, n H=−0.97±0.1). Data points are mean±s.e.m. of 3–6 measurements. Full size image Indeed, Zn 2+ dose-dependently inhibited 100 μM ATP (saturating)-induced channel activation of rP2X4 V288H/T211H (IC 50 , the concentration of Zn 2+ yielding half of the inhibition=25.6±5.7 μM; n H=−0.97±0.1; Fig. 4b,c ). As control, Zn 2+ (200 μM, saturating) slightly potentiated rather than inhibited ATP currents of wild-type rP2X4 receptors as well as the single histidine mutant r T211H ( Fig. 4b,c ). Unexpectedly, Zn 2+ inhibited ATP currents of another single histidine mutant r V288H ( Fig. 4c ), indicating that the native histidine residues or backbone atoms could form a metal site together with r V288H. Indeed, the double-mutant r V288H/H286A abolished Zn 2+ -mediated inhibition. However, Zn 2+ inhibited ATP currents of triple mutants r V288H/T211H/H286A and r V288H/T211H/H140A, and the quadruple mutant r V288H/T211H/H140A/H286A ( Fig. 4c ), suggesting that the Zn 2+ -mediated blockage in r V288H/T211H was not relying on nearby native histidine residues (H140 and H286). Taking advantage of lacking native histidine residue at the identical position of r H286 and r H140 in zfP2X4 ( Supplementary Fig. 4c ), we further tested the effect of Zn 2+ on ATP currents of zfP2X4 V291H/S214H . Zn 2+ inhibited ATP currents of zf V291H/S214H but not of single mutants zf V291H and zf V214H, as well as the wild-type zfP2X4 ( Supplementary Fig. 4d,e ), confirming the idea that an interdomain metal bridge between LF and DF is sufficient to inhibit ATP currents of P2X4 receptors. Therefore, an engineered zinc bridge between LF and DF domains is capable of inhibiting the channel activation of P2X4 receptors by preventing the relative motion of LF and DF domains. Altered hydrophobic interactions between LF and DF domains To further address the mechanism underlying ATP-binding-induced coordinated motions of LF and DF domains, the ATP-binding mode at the very beginning of ATP contacting with resting zfP2X4 was established by in silico docking ( Supplementary Fig. 5a ). A superposition and comparison of the resting and open structures of zfP2X4 ( Supplementary Fig. 5c ), both with bound ATP, showed that the side chains of key residues K70, K72, R143 and T189 directly interacting with ATP underwent conformational changes during channel gating ( Supplementary Fig. 5c ). In contrast, the conformation of other residues R298, K316, N296, I232 and L191 had no significant changes during channel gating ( Supplementary Fig. 5c ). Notably, some partially conserved hydrophobic residues ( Supplementary Fig. 4a ) within the P2X receptor family, such as zf L217, zf I208, zf V291 and aliphatic side chain of zf K193 interacting with each other via hydrophobic interactions, underwent conformational changes passing from resting to open state ( Fig. 5a ). The dihedral angles of χ 2 (along C β –C γ ) of zf K193 and zf L217 experienced mild changes during transformation from resting to open states ( χ 2 zf K193 =−178 o versus −171 o ; χ 2− zf L217 =−71.7 o versus −60.9 o , resting state versus open state), whereas the χ 1 angle (along C α –C β ) of zf V291 and χ 2 angle of zf L208 underwent marked alterations (χ 1 − zf V291=−75° versus −170°; χ 2- zf I208 =173.2° versus −85.8°, resting state versus open state). The free-energy profiles for those interaction pairs were reconstructed by metadynamics, ‘a powerful algorithm that can be used for both reconstructing the free energy and accelerating rare events in systems described by complex Hamiltonians’ [19] , where the dihedral angles of those four residues mentioned above were defined as the collective variables (CVs). The lowest free-energy paths (red arrows) plotted onto free-energy profiles passing from resting to open states revealed many ‘transition’ states (blue arrows) corresponding to higher potential energy along transition process, during which the bound ATP may help to overcome these energy barriers. Most importantly, those four residues were located at the interface between LF and DF domains ( Fig. 5a ), implying their possible roles in ATP-binding-induced coordinated movements of those two domains. 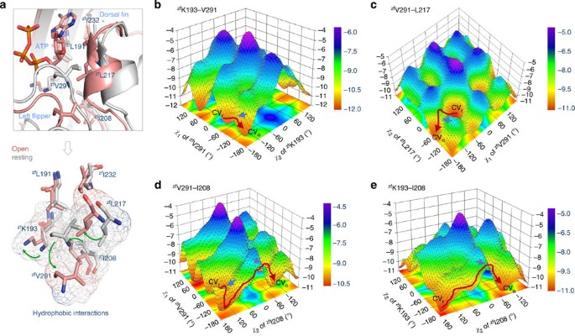Figure 5: Alterations in interdomain hydrophobic interactions between LF and DF domains after ATP-binding. (a) A superposition of the resting (grey, PDB ID code 3H9V) and open (pink, PDB ID code 4DW1) structures of zfP2X4 (upper panel) to show the alterations of hydrophobic interactions among I208, L217, V291 and K193 (displayed in sticks and surrounded with mesh for emphasis in lower panel). Green arrows denote the movement of key residues from the closed state to the ATP-bound open state. (b–e) Three-dimensional projection of the free-energy (kcal mol−1) surface showing the lowest free-energy paths passing from resting to open states of zfP2X4 receptors.CVrandCVoindicate the CVs at the resting and open states, respectively. The red arrows depict the lowest free-energy paths passing from resting to open states; the blue arrows denote the ‘transition’ state corresponding to higher potential energy along transition process. Similar results were obtained in two other independent metadynamics runs for each interaction pair. Figure 5: Alterations in interdomain hydrophobic interactions between LF and DF domains after ATP-binding. ( a ) A superposition of the resting (grey, PDB ID code 3H9V) and open (pink, PDB ID code 4DW1) structures of zfP2X4 (upper panel) to show the alterations of hydrophobic interactions among I208, L217, V291 and K193 (displayed in sticks and surrounded with mesh for emphasis in lower panel). Green arrows denote the movement of key residues from the closed state to the ATP-bound open state. ( b – e ) Three-dimensional projection of the free-energy (kcal mol −1 ) surface showing the lowest free-energy paths passing from resting to open states of zfP2X4 receptors. CV r and CV o indicate the CVs at the resting and open states, respectively. The red arrows depict the lowest free-energy paths passing from resting to open states; the blue arrows denote the ‘transition’ state corresponding to higher potential energy along transition process. Similar results were obtained in two other independent metadynamics runs for each interaction pair. Full size image To examine the involvement of those hydrophobic residues in the movements of LF and DF domains, another set of normal MD simulation was used, in which the ATP-binding mode at the very beginning of ATP contacting with the resting zfP2X4 was set as the initial structure to replay the process of ATP-binding-induced coordinated movements of LF and DF domains. ATP made no contacts with side chains and main chains of zf K70, zf K72 and zf T189 at the initial ATP-bound zfP2X4 resting structure. However, as revealed by increased total number of H-bonds from 4 to 6–8 ( Supplementary Fig. 6a ), these contacts were quickly established or strengthened after 10 ns MD simulations. Furthermore, the N–O distance between zf K193 and the α-phosphate of ATP was shortened from 7.5 to 4.8 Å after 20 ns simulations, achieved by a long-distance electrostatic attraction ( Supplementary Fig. 6b ). In contrast, the zf K193– zf I208 distance made no significant changes ( Supplementary Fig. 6c ), indicating that the hydrophobic interaction between zf K193– zf I208 remained despite the change of the location of zf K193. Meanwhile, the distance of zf L217 (DF)-ATP was shortened from ~8 to 4.5–5.8 Å via hydrophobic interactions among the adenine base of ATP, DF and head domains after 20-ns simulations ( Supplementary Fig. 6d ), so were the distances of zf V291 (LF)– zf I208 and zf L217 (DF)– zf I208 ( Supplementary Fig. 6e,f ). Along with those structural rearrangements, zf V291, located on LF domain, was repelled by the ribose of ATP ( Supplementary Fig. 6g ). Most importantly, along with those allosteric changes, the relative motions between LF and DF domains comparable to the open crystal structure were observed ( Supplementary Fig. 6h ), especially for the LF domain, indicating that alterations in hydrophobic interactions of zf V291, zf I208, zf L217 and zf K193 were correlated well with ATP-binding-induced coordinated motions of those two domains. Results of the lowest free-energy paths passing from resting to open states ( Fig. 5b–e ) and normal MD simulations also disclosed other details for bound-ATP-induced structural rearrangements of those four residues during channel gating. The transition paths revealed that the transition of the dihedral angle χ 1 of zf V291 from −75°to −170° has priority over changes in dihedral angles of zf K193, zf I208 and zf L217 ( Fig. 5b–d ) in the process of passing from resting to open state, especially for zf I208 ( Fig. 5d ). Indeed, at the very beginning (3 ns) of normal MD simulations on closed zfP2X4 complexes with pre-docked ATP, we observed bound-ATP-induced changes of χ 1 angle of zf V291 from −75° to −170°, whereas only mild changes occurred in the χ 2 angles of zf K193, zf I208 and zf L217 ( Supplementary Fig. 7a ). The pre-docked ATP in closed zfP2X4 was also able to stabilize the χ 1 angle of zf V291 at −170° during normal MD simulations ( Supplementary Fig. 7b ). Those data indicated that the bound-ATP-induced changes of χ 1 angle of zf V291 and the following repelling action on zf V291 caused conformational changes of zf K193, zf I208 and zf L217. Those allosteric changes led to final relative motions between LF and DF domains. Role of hydrophobic interactions between LF and DF domains As illustrated in Fig. 6a , ATP-binding-induced coordinated movements of LF and DF domains may be achieved by the repelling of zf V291 (LF) and the closing movements of zf K193, zf L217 (DF) and zf I208 (DF) to ATP. In this process, the changed interactions of zf V291, zf I208, zf L217 and the aliphatic chain of zf K193 are essential for the relative motions between LF and DF domains. Indeed, mutations on r K190 of rP2X4 (corresponding to zf K193 of zfP2X4), r K190A, r K190L and r K190F, which lacked the basic group ( r K190L), or had either smaller ( r K190A) or bulkier ( r K190F) size of the aliphatic side chain, strongly reduced the saturated ATP-induced maximal current of rP2X4 ( Fig. 6b,c ). These reduced activities may result from blocking the r K190-ATP interaction and the altered entire architecture of the hydrophobic interactions between LF and DF domains. Meanwhile, mutations in other three residues r I205, r L214 and r V288 of rP2X4 (corresponding to zf I208, zf L217 and zf V291 of zfP2X4, respectively) involved in hydrophobic interactions contributing to DF and LF domains coordinated movements, r I205G, r I205C, r I205D, r I205W, r L214A, r L214C, r L214W, r V288G, r V288A, r V288C and r V288F, with smaller or bulkier size of side chains, or with an introduction of hydrophilic side chain to break the hydrophobic interaction, also significantly diminished or fully abolished the maximal currents of rP2X4 ( Fig. 6b,c ). In contrast, consistent with the observation that zf L191, zf I232, zf L209 and zf I212, close to zf I208, zf L217, zf V291 and zf K193, displayed no significant conformational changes during the coordinated movements of LF and DF domains ( Fig. 6a ), mutations on the corresponding residues of rP2X4, r L188F, r L206A, r I209G, r I229A and r I229F only partially reduced the maximal current of rP2X4 ( Fig. 6b,c ). 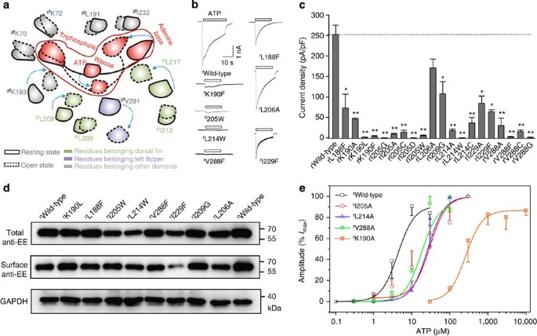Figure 6: ATP-binding-evoked alterations in interdomain hydrophobic interactions is crucial for P2X4 receptor activation. (a) Illustrations of bound-ATP-evoked alterations in interdomain hydrophobic interactions between LF and DF domains. Dotted arrows indicate the movements of key residues and ATP after ATP-binding. (b) Representative current traces showing maximal amplitude of currents caused by saturated ATP (1–1.5 mM forrK190F,rI205W,rL214W,rI229F andrV288F; 100 μM for WT,rL188F andrL206A). (c) Pooled data for maximal current activated by saturated ATP for mutations of the residues involved in interdomain interactions (means±s.e.m.,n=5–31). *P<0.05; **P<0.01 versus WT (dashed line), Student’st-test. (d) Representative western blotting illustrating effects of various mutants on the cell surface expression of rP2X4. Similar results were obtained in three other independent experiments. (e) Effect of mutations on ATP-sensitivity of rP2X4. The solid line is a fit of the Hill equation to the pH-dependent activation. Each point represents the mean±s.e.m. of 3–6 measurements. Figure 6: ATP-binding-evoked alterations in interdomain hydrophobic interactions is crucial for P2X4 receptor activation. ( a ) Illustrations of bound-ATP-evoked alterations in interdomain hydrophobic interactions between LF and DF domains. Dotted arrows indicate the movements of key residues and ATP after ATP-binding. ( b ) Representative current traces showing maximal amplitude of currents caused by saturated ATP (1–1.5 mM for r K190F, r I205W, r L214W, r I229F and r V288F; 100 μM for WT, r L188F and r L206A). ( c ) Pooled data for maximal current activated by saturated ATP for mutations of the residues involved in interdomain interactions (means±s.e.m., n =5–31). * P <0.05; ** P <0.01 versus WT (dashed line), Student’s t -test. ( d ) Representative western blotting illustrating effects of various mutants on the cell surface expression of rP2X4. Similar results were obtained in three other independent experiments. ( e ) Effect of mutations on ATP-sensitivity of rP2X4. The solid line is a fit of the Hill equation to the pH-dependent activation. Each point represents the mean±s.e.m. of 3–6 measurements. Full size image In addition, the surface expression levels of both the functional or loss-of-function mutants of rP2X4 exhibited no pronounced changes when compared with that of the wild-type rP2X4 receptor, except for r I229F ( Fig. 6d ), indicating their critical role in channel gating rather than surface expression. Furthermore, alanine substitutions on the r I205, r L214 and r V288 led to significant reduction of maximal currents of rP2X4 ( Fig. 6c ), but only slightly decreased their apparent affinities of ATP (EC 50 =13.8±4.1, 22.5±6.3, 12.9±1.3 μM for r I205A, r L214A and r V288A, n =3–4, respectively) when compared with that of wild-type rP2X4 (EC 50 =7.34±2.8 μM, n =4) ( Fig. 6e ). Meanwhile, alanine replacement on r K190 led to a significantly increased EC 50 value of r K190A (233±69 μM, n =4, ~30-fold decreased the ATP-sensitivity of rP2X4) possibly because of its direct electrostatic contact with ATP, indicating its important role in ATP-sensing. Notwithstanding, the contribution of r K190 in ATP-sensing is much weaker than other key residues involved in directly contacting with ATP [20] . Our data revealed that the residues involved in ATP-binding-induced altered interdomain hydrophobic interactions are essential for channel activation of rP2X4 receptor rather than the surface expression and the ATP-sensing, at least for r I205, r L214 and r V288. Here we identify the indispensable role of relative motions between the LF and DF domains in channel gating of P2X4 receptors using a combination of computational and experimental studies. All the molecular modelling was done on the crystal structure of zfP2X4, whereas the mutagenesis was done with the rP2X4. This is because ATP is not very potent at activating the zebra fish receptor expressed in HEK cells. Despite the difference in P2X sequences among species, the number of residues that form the LF, DF and head domains are the same between rP2X4 and zfP2X4 receptors. The key hydrophobic residues located at the interface of the LF and DF domains are also highly conserved between rP2X4 and zfP2X4 ( Supplementary Fig. 4a ). As a result, mutations of those residues in zfP2X4 significantly reduced ATP (1 mM)-induced currents ( Supplementary Fig. 4f,g ). A metal bridge between the LF ( zf V291H) and DF ( zf V214H) domains also inhibited ATP currents of zfP2X4 ( Supplementary Fig. 4d,e ). All this evidence suggests that the same mechanism is responsible for coupling LF and DF’s dynamics with channel gating in rP2X4 and zfP2X4. The molecular modelling together with mutagenesis in our work revealed that ATP-binding-induced alterations in interdomain hydrophobic interactions and the concomitant coordinated motions of the LF and DF domains are allosteric changes essential for the channel activation of P2X4 receptors. Those conformational changes are distinct from previously identified allosteric events essential for channel activations, such as the downward motion of cysteine-rich head domain, tightening of the ATP-binding site jaw and the upper vestibule expansions [5] , [6] , [8] , [9] . As revealed by the spontaneous closure of the ATP-binding site jaw ( Fig. 1b ) as well as the upper vestibule expansion in the absence of ATP-binding during MD simulation ( Fig. 1c ), inherent dynamics has a dominant role in determining those allosteric events. However, MD simulations together with NMA analysis revealed that the bound ATP may break the inherent dynamics of LF and DF domains, suggesting that the relative motions between the LF and DF domains evoked by bound ATP may act as a conformational switch to mediate the channel activation of P2X4 receptors. This assumption was supported by the findings that the engineered disulphide crosslinking and Zn 2+ bridge between the LF and DF domains significantly influenced the activation of P2X4 receptors ( Figs 3 and 4 ). Although ATP-binding-induced relative motions between LF and DF domains are allosteric events indispensable for the channel activation of P2X4 receptors, the mechanism underlying this process still remains unclear. This may be because of the following possible reasons: first, the hydrophobic interactions of the LF and DF domains at the resting state may develop an energy barrier to prevent channel activations. The downward motion of LF domain induced by ATP-binding is essential for overcoming of this energy barrier and favours downstream allosteric changes coupling to channel activations of P2X4 receptor. Second, given the rigidity of the body domain, like a ‘lever’, the ATP-bound crystal structure reveals a ‘lever’ mechanism that link binding site closure to iris-like pore opening [5] , [21] . The DF domain is structurally coupled to this ‘lever’. The upward movement of the DF domain induced by hydrophobic interactions among DF and head domains may drive the expanding motion of the lower body domain (‘lever arm’). Third, LF domain is located at the intersubunit interface of two lower body domains. One side of the LF domain is structurally coupled to the body domain of one subunit, and the other side contacts with the body domain and DF domain of another subunit. Bound ATP-evoked altered hydrophobic interactions between the LF and DF domains, and the downward motion of the LF domain might favour outward flexing of those two lower body domains and facilitate the final opening of P2X4 receptors. Indeed, during MD simulations on the closed zfP2X4 complexes with pre-docked ATP, we have observed a mild pore dilation in the TM regions, which became more obvious along with the relative motions of the LF and DF domains ( Supplementary Fig. 8a,c ) when compared with the simulations on receptors in the absence of pre-docked ATP ( Supplementary Fig. 8c ). The obvious expansion of central vestibule (formed by lower body domains of three subunits) and upward movements of linker regions ( Supplementary Figs 1a and 8a–c ) resulted in outward movements of TM1 and TM2 ( Supplementary Fig. 8a ). Those allosteric changes led to a final pore dilation of zfP2X4, consistent with the observation in the open crystal structure ( Supplementary Fig. 8d ). In contrast, during MD simulations on the closed structure without pre-docked ATP, only a mild spontaneous expansion of central vestibule and the upward movements of linker regions were detected ( Supplementary Fig. 8e ). Therefore, the rigid lower body domains and linker regions may enable the coupling of the relative motions between LF and DF domains and the outward motions of the TM helixes. Finally, taking into consideration the crucial role of relative motions between LF and DF in channel gating of P2X4 receptors, the cleft existing among LF, DF and head domains provides an opportunity to develop new subtype-specific small molecules interacting with this site ( Supplementary Fig. 4b ). We proposed that a bound small molecule at this site may potentially block the activation of P2X receptors. Here are some hints on this hypothesis: first:, the bound small molecules at this site may stabilize the interactions between LF and DF domains, and curb their relative motions via contacts with the hydrophobic residues in the interface of these two domains, such as r V288, r I205, r L214 and their nearby residues. Those interactions will increase the energy barrier for the channel gating. Second, as revealed by the crystal structures of zfP2X4 (refs 4 , 5 ), the bound ATP makes contacts with residues located at the interface of the LF, DF and head domain via weak hydrophobic interactions ( Supplementary Fig. 4b ). The bound small molecules occupying this cleft/cavity may compete with the ATP. Finally, the residues exposed to this cleft/cavity are not conserved throughout the P2X receptor family ( Supplementary Fig. 4b,c ), providing a possibility to develop subunit-specific blockers of P2X receptors. Thus, the identification of open-related movements of LF and DF domains together with identified allosteric changes of head domain will help to develop subunit-specific blockers of P2X receptors. In summary, ATP-binding-evoked P2X channel gating is a very precise and complex process, including allosteric conformational changes in head, LF, DF, body and TM domains. ATP-binding has roles in tightening the binding site and coordinating the motion of whole receptors, which leads to the reduction of energy barrier and the subsequent channel activation. The identification of open-related movements of those domains would enable the evaluation of new strategies aiming at developing new subtype-specific blockers of P2X receptors. Molecular biology ATP, ZnCl 2 and most of other drugs were purchased from Sigma (St Louis, MO, USA). The plasmid pcDNA3-rP2X4 is the gift from Drs Alan North and Lin-Hua Jiang, and the cDNA of zfP2X4.1 obtained from Dr Eric Gouaux was subcloned into the pcDNA3 vector (all the primers that have been used see Supplementary Table 1 ). Each mutant was generated with a QuikChange mutagenesis kit. Individual mutations were verified by DNA sequencing. All constructs were expressed in HEK-293 cells. HEK-293 cells were cultured in DMEM medium at 37 °C in a humidified atmosphere of 5% CO 2 and 95% air. Transfections of plasmids were performed using Hilymax (Dojindo Laboratories, Kumamoto, Japan) following the manufacturer’s recommendation. Electrophysiological measurements were performed 24–48 h after transfection as we described previously [22] . Electrophysiology The electrophysiological recordings were performed using the conventional whole-cell configuration under the voltage clamp at room temperature (23±2 ° C) as our previous description [14] , [22] . In brief, patch pipettes were pulled from glass capillaries on a two-stage puller (PC-10, Narishige). The resistance between the recording electrode was filled with pipette solution and the reference electrode was 3–5 MΩ. Membrane currents were measured using an Axon patch 200B patch clamp amplifier (Molecular Devices) and were filtered at 2 kHz using low-pass Bessel filter. All currents were sampled and analysed using a Digidata 1440 interface and a computer running the Clampex and Clamp-fit 10.0 software (Molecular Devices). The bath solution contained 150 mM NaCl, 5 mM KCl, 10 mM glucose, 2 mM CaCl 2 .2H 2 O, 10 mM HEPES and 1 mM MgCl 2 .6H 2 O; the pH was adjusted to 7.35. Patch electrodes were filled with solution containing 30 mM NaCl, 120 mM KCl, 1 mM MgCl 2 .6H 2 O, 0.1 mM CaCl 2 .2H 2 O and 5 mM EGTA; the pH was adjusted to 7.35. In most experiments, 70–90% of the series resistance was compensated. The membrane potential was held at −60 mV throughout the experiment under voltage-clamp conditions. ATP solutions were prepared in batch buffer for 2 h at most and applied using a fast pressure-driven microperfusion system (OctaFlow08P, computer controlled, ALA Scientific Instruments). Responses were normalized to cell membrane capacitance. Dose–response data were collected from recording of a range of ATP concentrations buffer, and the corresponding currents were normalized to the highest current amplitude; ATP-gated currents were recorded after regular 3 s ATP application every 2 min. For higher ATP concentrations (>10 μM), the pulses were spaced up to 5–15 min to avoid receptor desensitization. To abolish the rundown of currents in multiple-dose applications of ATP, the amphotericin-perforated patch clamp [23] was also used for current recordings of dose-dependent activations of rP2X4 V288C/T211C in initial absence and the subsequent presence of reducing agents, as well as the dose-dependent inhibition of Zn 2+ on ATP currents of rP2X4 V288H/T211H . During this procedure, ATP-gated currents were recorded after regular 15–20 s ATP application every 8 min to avoid receptor desensitization. Cell surface biotinylation and western blotting analysis Cell surface biotinylation and western blotting were performed as we previously described [24] . In brief, the HEK-293 cells transfected with rP2X4 or its mutants were washed in chilled PBS +/+ , and then incubated with sulfo-NHS-LC-biotin. The reaction was terminated by further incubating the cells with glycine in PBS. The cells were then collected and lysed with RIPA buffer. Biotinylated proteins were separated from the intracellular protein fraction using agarose resin linked to NeutrAvidin by incubation overnight and subsequent centrifugation. The resins were then washed and bound proteins were eluted with the boiling SDS sample buffer, while 10% of the volume of the supernatant was diluted and used as the total protein fraction. Protein samples from biotinylation assay were analysed by western blotting. The samples were separated by SDS-PAGE and transferred to a polyvinylidene difluoride (PVDF) membrane. The membrane was incubated overnight at 4 °C with anti-EE-tag (1:1,000; Abcam, catalogue number ab40767) or anti-GAPDH (1:1,000; Sungene Biotech, catalogue number KM9002) antibodies, followed by appropriate HRP-conjugated secondary antibodies for EE-tag (25 °C, 1 h, 1:1,000; Goat-Rabbit IgG(HtL)-HRP; Sungene Biotech, catalogue number: LK2001) or GAPDH (25 °C, 1 h, 1:3,000, Goat-Mouse IgG(HtL)-HRP; Sungene Biotech, catalogue number LK2003) and finally visualized using an ECL solution (Thermo) and exposure with ImageQuant RT ECL system (GE Healthcare, USA) for 1–3 min. All western blots and gels are accompanied by the locations of molecular weight markers (Thermo PageRuler Prestained Protein Ladder 10–170 kDa, catalogue number 26617) ( Supplementary Fig. 9 ). Protein dynamics simulations All MD simulations were performed by using the programme DESMOND 3.0 (ref. 25 ) with constant number of particles, pressure and temperature (NPT) and periodic boundary conditions (10 Å buffer distance to each dimension of the simulation box), which uses a particular ‘neutral territory’ method called the midpoint method to efficiently exploit a high degree of computational parallelism. A default OPLS_2005 force field, following the functional form of the OPLS-AA family of force fields with additional stretch, bend and torsional parameters for better coverage of ligand functional groups [26] , was used for the protein and ligand molecules. The energy-minimized structures of zfP2X4 by DESMOND 3.0 at the resting (PDB ID code 3H9V) or the open state (PDB ID code 4DW1) were used as the starting structures for MD simulations. The ATP-binding mode at the resting state of zfP2X4 was established by Autodock 4.2 (ref. 27 ); the pose with similar features as the open crystal structure of zfP2X4 was minimized by DESMOND 3.0 and was selected as the initial structure in the ATP-resting zfP2X4 complexes simulation system. A large dimyristoylphosphatidylcholine bilayer consisting of 253 membrane molecules, was constructed to generate a suitable membrane system in which the TM domain of the zfP2X4 could be embedded. The protein/dimyristoylphosphatidylcholine system was then solvated in a bath of simple point charge water molecules. Counter ions were subsequently added to compensate for the net negative charge of the system. NaCl (150 mM) was added into the simulation box that represents background salt at physiological conditions. To maintain the system at a constant temperature of 300 K, the Berendsen algorithm was applied to couple protein and other molecules separately with a coupling time of 0.1 ps. All of the bond lengths including hydrogen atoms were constrained by the Linear Constraint Solver algorithm. Electrostatic interactions between charged groups at a distance <9 Å were calculated explicitly; long range electrostatic interactions were calculated using the smoothed particle mesh Ewald method. All of the MD simulations were run on the DAWNING TC2600 (with 200 AMD Opteron 8374HE CPUs). Preparation, analysis and visualization were performed on a 12-CPU CORE DELL T7500 graphic working station. The pore radius was measured by using the programme HOLE [28] . PCA and NMA analysis were conducted by using the programme ProDy 1.1 (ref. 29 ). PCA modes of zfP2X4 dynamics were obtained by essential dynamics analysis of snapshots of MD simulations of zfP2X4. Low-frequency NMA modes of apo zfP2X4 were predicted by Anisotropic Network Model) Module of Prody 1.1 (ref. 29 ). These two measurements were performed using the default Prody parameters. Ten modes were generated in both NMA and PCA analysis by Prody. The modes with a tendency of closing the ATP-binding site jaw were selected. Models of zfP2X4 V291C/214C and zfP2X4 V291H/S214H The structures of the closed (PDB ID code 3H9V) and open (PDB ID code 4DW1) zfP2X4 receptors were taken as the templates to construct the zfP2X4 V291C/214C and zfP2X4 V291H/S214H models with the programme MODELLER [30] . For the disulphide bridge construction, the disulphide bond between two cysteine residues C291 and C214 was auto-connected by MODELLER [30] . Zinc-bridge model was constructed according to previous procedure [8] using MODELLER. In brief, for zinc-binding site reconstructions, a distance constrain (2.0–2.2 Å) was added between zinc and the NE2 atom of histidines and then was minimized by DESMOND 3.0 with OPLS_2005 force field [31] . The resulting two models of zfP2X4 V291C/214C and zfP2X4 V291H/S214H were further optimized by 1.2-ns MD simulations using programme DESMOND 3.0 with OPLS_2005 force field [31] . After such timescale of MD simulations, various parameters of zinc and disulphide bridges, including distances between atoms, bond angles and dihedral angles were very closing to those obtained by analysis of crystals. Metadynamics analysis Metadynamics [19] , [32] , [33] is a technique in which the potential for one or more chosen variables is modified by periodically adding a repulsive potential of Gaussian shape at the location given by particular values of the variables. In the present study, all metadynamics analysis were conducted by programme DESMOND 3.0 (ref. 25 ) under NPT and periodic boundary conditions using the default parameters at constant temperature (300 K) and pressure (1 bar) by using the Berendsen coupling scheme with one temperature group. All simulations used the OPLS_2005 force field for proteins and ions and the simple point charge model for water. The dihedral angles of side chain of key residues were set up as CVs. To set up CVs, four carbon atoms (C α , C β , C γ and C δ for zf K193, zf I208 and zf L217, and C α , C β , C γ and one backbone carbon atom for zf V291) were selected to define the dihedral angles. The parameters for height, width of the Gaussian, and the interval were set to 0.03 kcal mol −1 , 5° and 0.09 ps, respectively. All metadynamics runs were protracted for ~20,000 ps until they showed a free diffusivity along the defined CVs. This criteria was chosen according to the guidelines of assessing the accuracy of metadynamics runs [33] . The sum of the Gaussians and the free-energy surface were generated by METADYNAMICS ANALYSIS tools of DESMOMD 3.0. Data analysis The results are expressed as the means±s.e.m. Statistical comparisons were made using the t -test, where P <0.05 (*) or P <0.01 (**) was considered significant. Concentration–response relationships for ATP activation of wild-type or mutated channels were obtained by measuring currents in response to different concentrations of ATP, and all of the results used to generate a concentration–response relationship were from the same group. The data were fit to the Hill equation: I / I max =1/[1+(EC 50 /[ATP]) n ], where I is the normalized current at a given concentration of ATP, I max is the maximum normalized current, EC 50 is the concentration of ATP yielding a current that is half of the maximum and n is the Hill coefficient. How to cite this article: Zhao, W.-S. et al. Relative motions between left flipper and dorsal fin domains favour P2X4 receptor activation. Nat. Commun. 5:4189 doi: 10.1038/ncomms5189 (2014).